Epitaxial growth of inch-scale single-crystal transition metal dichalcogenides through the patching of unidirectionally orientated ribbons Two-dimensional (2D) semiconductors, especially transition metal dichalcogenides (TMDs), have been envisioned as promising candidates in extending Moore’s law. To achieve this, the controllable growth of wafer-scale TMDs single crystals or periodic single-crystal patterns are fundamental issues. Herein, we present a universal route for synthesizing arrays of unidirectionally orientated monolayer TMDs ribbons (e.g., MoS 2 , WS 2 , MoSe 2 , WSe 2 , MoS x Se 2-x ), by using the step edges of high-miller-index Au facets as templates. Density functional theory calculations regarding the growth kinetics of specific edges have been performed to reveal the morphological transition from triangular domains to patterned ribbons. More intriguingly, we find that, the uniformly aligned TMDs ribbons can merge into single-crystal films through a one-dimensional edge epitaxial growth mode. This work hereby puts forward an alternative pathway for the direct synthesis of inch-scale uniform monolayer TMDs single-crystals or patterned ribbons, which should promote their applications as channel materials in high-performance electronics or other fields. Two-dimensional (2D) semiconducting transition metal dichalcogenides (TMDs) have attracted tremendous interest for their broad-range applications in electronics, optoelectronics, catalysis, etc. [1] , [2] , [3] . The morphology or dimensionality of TMDs is a critical factor to determine their physical properties. For instance, one-dimension (1D) monolayer MoS 2 ribbon is predicted to possess novel properties such as metallic edge states [4] , 1D confined plasmons [5] , ferromagnetic behaviors [6] , etc. Besides, it can present improved catalytic property in hydrogen evolution reaction (HER) due to the abundant active edge sites [7] , and more importantly, maintained high carrier mobility [8] . So far, the fabrication of monolayer TMDs ribbons has largely depended on micro-nanofabrication approaches, by using electron beam or optical lithography patterning techniques [9] . However, these top-down methods are evidently tedious and usually need to start with large-area uniform continuous films or crystals. Recently, several strategies have been developed for the direct synthesis of monolayer TMDs ribbons [10] , such as Na-Mo-O droplets driven growth on NaCl single crystals [11] , substrate-directed synthesis on phosphine pre-treated Si(001) substrates [12] , as well as ledge-directed epitaxy on β-Ga 2 O 3 (100) [13] . These strategies have individually achieved the control of their thickness, orientation and dimensionality, nevertheless, the synthesis of TMDs ribbons possessing all the above advantages has not been realized. Wafer-scale monolayer TMDs single crystals, characterized by intrinsically high crystallinity and extremely uniform property, have long been pursued. However, due to the non-centrosymmetric structures of TMDs, antiparallel domains and twin boundaries usually evolved on most growth substrates [14] , [15] , [16] , similar to those encountered in the preparation of h -BN. Lately, wafer-scale growth of monolayer h -BN single crystal was achieved by using liquid Au as substrate via the self-collimation of circular h -BN grains [17] . Wafer-scale monolayer h -BN single crystals were also realized on Cu(110) [18] and Cu(111) [19] substrates, where the nucleation and growth of h -BN domains were dominantly guided by the substrate-step edges. Very recently, our group realized the epitaxial growth of inch-scale monolayer MoS 2 single crystals on Au(111) films [20] , demonstrating the potential for the unidirectionally oriented growth of TMDs grains. Despite these achievements, the successful attempts regarding the growth of wafer-scale monolayer TMDs single crystals on Au substrates remain very limited [21] , [22] . Meanwhile, the step-edge-guided growth of single-crystal TMDs has also been explored on insulating sapphire substrates [23] , [24] , [25] , [26] . Particularly, inch-scale single-crystal MoS 2 and WS 2 monolayers have been achieved on C-A and A plane sapphire substrates, in which the nucleation of MoS 2 and WS 2 are along the <10 \(\bar{1}\) 0> step edges of sapphire, further proving the effect of step edges on the alignment of TMDs domains. However, the direction of the step edge on sapphire is highly dependent on the miscut direction, and it is rather difficult to maintain a fixed cutting angle with such a high accuracy (e.g.,1°) over an inch scale. Herein, we design a substrate-step templated growth strategy for synthesizing large-area uniform, unidirectionally aligned, monolayer single-crystal TMDs ribbons, by using the step edges of vicinal Au(111) single crystals as growth fronts. The superiorities of this route are summarized as follows: (1) the uniformly oriented step edges on high-index Au facets can trigger the anisotropic growth of TMDs, and direct the alignment of the resulted monolayer ribbons; (2) the chemical inertness of Au substrate to chalcogen precursor makes it a universal template for synthesizing various monolayer TMDs ribbons (e.g., MoS 2 , WS 2 , MoSe 2 , WSe 2 ); (3) different from the growth on insulating substrates, the monolayer TMDs grown on Au metals are featured with relatively strong interface coupling, which can be another parameter for mediating the van der Waals epitaxial growth of 2D layered materials toward wafer-scale single crystals; (4) the synergistic effect of substrate-step-edge guided 1D epitaxy, combined with substrate-lattice-match directed 2D epitaxy modes are expected to direct the epitaxial growth of single-crystal TMDs monolayers. This work is expected to offer an alternative strategy for the synthesis of monolayer patterned TMDs ribbons or wafer-scale single-crystal films. The practical applications of the dimension controllable monolayer materials (ribbons or films) will also be demonstrated in more versatile fields, e.g., as channel materials in high-performance electronic devices and as catalysts in HER. Theoretical calculations for the evolution of monolayer TMDs ribbons To initialize the growth of monolayer MoS 2 ribbons, it is a general route to introduce anisotropic template with broken symmetry, e.g., by introducing substrate steps [27] . Such a substrate-template-directed synthesis strategy has previously been used for the growth of 1D GaN [28] , graphene [29] , and MoS 2 nanowires [30] . In our experiment, a series of high-miller-index Au facets vicinal to (111) with bunched atomic steps were selected as growth templates, as obtained by melting and resolidifying Au foils on W templates (see Methods for more details). As reported previously, the types of the MoS 2 terminated edges were quite different for 1D stripes and 2D triangles, i.e., Mo-zigzag (Mo-zz)/S-zigzag (S-zz) edges and Mo-zz edges, respectively, as characterized by transmission electron microscope (TEM) in previous literatures [27] , [28] . Moreover, the edge type of monolayer MoS 2 achieved by the CVD growth process highly depended on the S/Mo ratio of precursors [31] , [32] , [33] , [34] . In this regard, the effect of S/Mo ratio should have a significant effect on the morphology of monolayer MoS 2 . To confirm this, CVD growth was executed on a representative Au(223) facet with MoO 3 and S as precursors (growth conditions: 750 °C for 3 min, Supplementary Fig. 1 ). When the mass ratio of S/Mo was set at 3:1, monolayer MoS 2 triangular domains were obtained (Fig. 1b ). As the S/Mo ratio decreased to 2:1, monolayer MoS 2 ribbons evolved under similar growth conditions (Fig. 1c ). X-ray photoemission spectroscopy (XPS) spectra confirmed the formation of MoS 2 compounds (Supplementary Fig. 2 ). Atomic force microscope (AFM) images of as-grown monolayer MoS 2 triangular domains and ribbons on Au substrates (Supplementary Fig. 3 ) clearly show that the edges of MoS 2 are usually aligned along the steps of Au substrates, providing straightforward evidence for the step-edge-guided growth mechanism. Nevertheless, further decreasing the S/Mo ratio to 1:1 led to the formation of irregularly shaped MoO x S 2− x crystals (Supplementary Fig. 4 ), probably due to the insufficient feeding of the S feedstock [30] . Fig. 1: Morphological evolution of monolayer MoS 2 from triangular to ribbon-like shaped domains. a Schematic illustration of the morphological evolution of MoS 2 . b , c SEM images of 2D monolayer MoS 2 triangles ( b ) and 1D ribbons ( c ) achieved at different S/Mo ratios. d Nucleation barrier (Δ E ) difference mapping between S-zz and Mo’-zz edges under different chemical potentials of Mo ( μ Mo ) and S ( μ S ). For the case of high μ S and low μ Mo (bottom right region), the nucleation barrier of S-zz is smaller than that of Mo’-zz edge (Δ E < 0), Mo’-zz edge is the dominating edge and the resulted MoS 2 flake presents a triangle shape. As μ S decreases (Δ E > 0, bottom left region), the S-zz edge becomes the dominating edge and the resulted MoS 2 flake shows quasi ribbon-like shape. e Schematic view showing the morphology variations of monolayer MoS 2 islands with decreasing the S/Mo ratio. Orange and yellow spheres indicate Mo and S atoms, while the orange and yellow lines represent Mo and S terminated edges, respectively. Full size image To further understand the role of S/Mo ratio in the morphological evolution of monolayer MoS 2 , density functional theory (DFT) calculations were then performed to simulate the MoS 2 growth on Au(111). The kinetic growth of MoS 2 can be analyzed by exploring the nucleation barriers of two dominating edges on Au(111) around <110> step during the atomic accretion process, i.e., S-zz and reconstructed Mo-terminated zigzag (Mo’-zz) edges due to their higher nucleation barriers than those of armchair, and Mo-zz (see details in Supplementary Figs. 5 ‒ 7 ). Using Mo atoms and S 2 dimers as the feeding units, the relative nucleation barriers (Δ E ) for these two edges under different chemical potentials of Mo and S (labeled as μ Mo and μ S , respectively) were calculated. For the case of high μ S and low μ Mo (bottom right in Fig. 1d ), the nucleation barriers of S-zz are smaller than that of Mo’-zz edges (Δ E < 0). Hereby, Mo-oriented edges should be prevalent in parallel with the evolution of triangular-shaped domains. As μ S decreases (Δ E > 0, bottom left in Fig. 1d ), the growth velocity of S-zz edge declines significantly, and S-zz edge becomes the dominating one. Following our previous results [20] , the minimum energy configuration corresponds to Mo-zz edges docking to Au <110> steps on the (111) surface. Thereby, the ribbons terminated with Mo-zz edges along the Au <110> steps (on one side) and terminated with free S-zz edges on the terraces (on the other side) should be more preferentially evolved. The schematic diagram in Fig. 1e depicts the shape evolutions of MoS 2 from triangles to isosceles trapezoid or quasi stripes with the change of S/Mo ratios. Controllable growth of uniformly aligned monolayer TMDs ribbons According to our theoretical calculations, the following mechanism is proposed for the formation of unidirectionally oriented monolayer MoS 2 ribbons. As schematically illustrated in Fig. 2a , MoS 2 species tend to first nucleate at the step edges on the high-miller-index Au facets, considering of the high binding energy between them. Under a relatively small S/Mo ratio, the growth rate of S-zz edge was slower than that of Mo-zz edge, inducing the formation of MoS 2 ribbons terminated by Mo-zz and S-zz edges on either side. Fig. 2: Universal growth of aligned monolayer TMDs ribbons along the step edges of Au(111) vicinal facets. a Schematic illustration of the growth of well-aligned monolayer MoS 2 ribbons along the step edges of vicinal Au(111) facets. The red, yellow, and blue spheres represent Mo, S, and O atoms, respectively, and the red arrows indicate the diffusion pathways of the active species. b , c Schematic side view and SEM image of aligned monolayer MoS 2 ribbons grown on Au(223) facet, respectively. d Representative Raman spectra of the edges (red) and centers (blue) of monolayer MoS 2 ribbons transferred on SiO 2 /Si substrates. e Raman mapping on the intensity of A 1g peak for a MoS 2 ribbon. The right panel is the magnified image of the white rectangle marked region in the left panel. The red and blue dots mark the edge and center positions of MoS 2 ribbon, respectively. a.u., arbitrary units. f , g Representative PL spectra of the edges (red) and centers (blue) of a MoS 2 ribbon and its PL mapping on the intensity of A peak. The right panel is the magnified image of the white rectangle marked region in the left panel. The red and blue dots in ( g ) mark the edge and center positions of MoS 2 ribbon, respectively. h , i Schematic side view and SEM image of monolayer MoS 2 ribbons grown on monolayer graphene covered Au(213) facet, respectively. j , k Schematic side view and SEM image of monolayer MoS x Se 2-x ribbons grown along the steps of Au(235) facet, respectively. Full size image As evidenced by scanning electron microscopy (SEM) images (Fig. 2c ), the derived MoS 2 ribbons are uniformly distributed on the Au(223) facet with unidirectional alignment. These monolayer MoS 2 ribbons present straight edges, totally distinct from the sawtooth-like edged nanoribbons stringed by triangular domains (grown on β-Ga 2 O 3 (100)) [13] . Moreover, the widths and lengths of the obtained MoS 2 ribbons are tunable within 20‒120 nm and 3‒30 um, respectively (Supplementary Fig. 8 ). 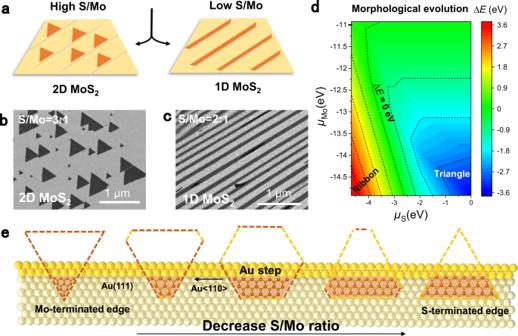Fig. 1: Morphological evolution of monolayer MoS2from triangular to ribbon-like shaped domains. aSchematic illustration of the morphological evolution of MoS2.b,cSEM images of 2D monolayer MoS2triangles (b) and 1D ribbons (c) achieved at different S/Mo ratios.dNucleation barrier (ΔE) difference mapping between S-zz and Mo’-zz edges under different chemical potentials of Mo (μMo) and S (μS). For the case of highμSand lowμMo(bottom right region), the nucleation barrier of S-zz is smaller than that of Mo’-zz edge (ΔE< 0), Mo’-zz edge is the dominating edge and the resulted MoS2flake presents a triangle shape. AsμSdecreases (ΔE> 0, bottom left region), the S-zz edge becomes the dominating edge and the resulted MoS2flake shows quasi ribbon-like shape.eSchematic view showing the morphology variations of monolayer MoS2islands with decreasing the S/Mo ratio. Orange and yellow spheres indicate Mo and S atoms, while the orange and yellow lines represent Mo and S terminated edges, respectively. Their aspect ratios (10 2 ‒10 3 ) are much larger than most of the TMDs ribbons reported previously (10‒10 2 ) [11] , [12] , [13] , [30] , [31] , [35] , [36] (Supplementary Table 1 ). AFM characterization of a typical MoS 2 ribbon shows a thickness of ~0.7 nm, again confirming its monolayer nature (Supplementary Fig. 9 ). Raman and photoluminescence (PL) spectra were then collected from the monolayer MoS 2 ribbons transferred on SiO 2 /Si substrates. The Raman characteristic peaks are fixed at ~386 cm −1 ( E 1 2g ) and 406 cm −1 ( A 1g ) (Fig. 2d ), with a frequency difference (Δ) ~20 cm −1 , justifying the monolayer nature of the MoS 2 ribbons [37] . However, the Raman intensity of the ribbon edge is slightly lower than that of the center region (Fig. 2e ), probably due to the reduced electron density at the ribbon edge. Meanwhile, the PL spectrum from the ribbon edge exhibits a blue-shifted peak (at ~677 nm) and lower intensity (Fig. 2g ) relative to the center region (at ~684 nm), which may arise from the strain at the ribbon edge [38] , [39] . More intriguingly, such step-edge-guided growth of monolayer MoS 2 ribbons was also realized on monolayer graphene or h -BN-covered vicinal Au(111) facets. As shown in Fig. 2i , well-aligned monolayer MoS 2 ribbons occurred on a monolayer graphene-coated Au(213) facet, as confirmed by the coexistence of characteristic Raman signals for monolayer MoS 2 , i.e., E 1 2g (~386 cm −1 ) and A 1g (~406 cm −1 ) peaks, and graphene on the same region (Supplementary Fig. 10 ). Besides, patterned monolayer MoS 2 ribbons were also achieved on the monolayer h -BN/Au(111) template (Supplementary Fig. 11 ). The compatibility of Au substrate with the growth of TMDs, graphene, and h -BN makes it possible to construct van der Waals heterostructures based on these 2D layered materials. Apart from monolayer MoS 2 , monolayer TMDs alloys ribbons, such as MoS x Se 2– x , were also achieved on an Au(235) facet by using mixed S and Se as chalcogen precursor (Fig. 2k ). Raman spectrum (inset of Fig. 6g ) shows two groups of characteristic peaks, in line with that of MoS 2 (at ~386 and 405 cm −1 ) and MoSe 2 (at ~270 cm −1 ), justifying the formation of MoS x Se 2– x compounds [40] . Given these facts, the substrate-step-edge guided growth route can be utilized as a universal pathway for the growth of TMDs ribbons and their alloys. Preparation of inch-scale high-miller-index Au single-crystal films The key point of this synthetic route relies on the preparation of anisotropic substrate of vicinal Au(111) single-crystal facets. To achieve this, Au foils on W templates were melted and resolidified at ~1100 °C and maintained for ~20 min. The schematic and photograph of a representative Au film (with a size of 3 cm × 3 cm) featured with Au(223) facet are presented in Fig. 3a, b , respectively. The facet surface was characterized by uniformly distributed, parallel bunched steps, as evidenced by the AFM image in Fig. 3c . X-ray diffraction (XRD) pattern of the as-prepared Au/W film shows the (111) peaks of Au film, and the (200) and (211) peaks of W foil (Fig. 3c ). Fig. 3: Preparation of inch-scale high-miller-index Au single-crystal films (Au(111) vicinal facets). a Schematic illustration of a high-index Au(223) facet. b Representative photography of the evolved Au(223) single-crystal film on the W template. c . XRD pattern of Au/W foils showing the evolution of single-crystal Au(111) film. Inset: AFM image of a single-crystal Au film with Au(223) facet. d Representative EBSD IPF maps of the as-prepared Au films, with crystal facets of (111), (223), (235), (456), (213), (346), (434), (345), respectively. The scale bars in all panels are 1 mm. e , f SEM images of the unidirectionally aligned monolayer MoS 2 ribbons evolved on single-crystal Au(456) ( e ) and Au(346) ( f ), respectively. Full size image However, due to the limited resolution of XRD, it is difficult to distinguish the exact miller-index of the Au facet. Further electron backscatter diffraction (EBSD) characterization reveals the evolution of such a single-crystal Au(223) facet (Fig. 3d ). Large-area EBSD maps collected on the whole sample surface show uniform color contrast and nearly undetectable angular variation (Supplementary Fig. 12 ), confirming the single crystallinity of the Au(223) facet. Notably, a series of single-crystal Au(111) vicinal facets were also achieved through the current annealing process, including (235), (213), (346), (456), etc. (Fig. 3d and Supplementary Fig. 13 ), as defined by the homogeneous color contrasts in the inverse pole figure maps. The derived high-miller-index Au facets belong to a category of facets vicinal to Au(111), which are composed of a regular succession of (111) terraces separated by monatomic steps. Notably, the appearance of a specific high-index facet is relatively random, as similarly proposed in the preparation of atomic sawtooth high-miller-index Au facets through different annealing processes [21] . Herein, the formation of the high-index facet is probably due to the close contact between Au liquid and W template at high temperature, in which the strain energy should be the driving force, rather than the surface energy for the formation of Au(111). This phenomenon was also reported in the preparation of high-miller-index single-crystal Cu foils, in which the stress on Cu foil was introduced by using graphite susceptor [41] . Notably, a variety of vicinal Au(111) facets, independent of the specific index (e.g., Au(456), Au(346)), were all proved to be capable of inducing the formation of monolayer MoS 2 ribbon arrays (Fig. 3e, f ). Besides, the as-grown monolayer MoS 2 ribbon presents a relatively high density on the high-miller-index Au facet with a high density of step (Supplementary Fig. 14 ). This provides an effective route for ribbon density regulation. Monolayer TMDs single-crystal films merged by 1D ribbons The lateral growth and merging behavior of monolayer TMDs ribbons were then investigated by deliberately increasing the coverage. As shown in Fig. 4b‒d , upon extending the growth time from 2, 4 to 6 min, monolayer MoS 2 ribbons with average widths of ~130 and ~190 nm, and continuous full-coverage MoS 2 film were achieved on the Au(223) facet steadily. In this regard, the growth should obey a step-flow growth mode, inducing the formation of single-crystal film through the merging of unidirectionally aligned grains. The single crystallinity of the monolayer film was first verified by low-energy electron diffraction (LEED) measurements. The obtained diffraction spots indicate the existence of MoS 2 on the high-index Au(223) stepped surface (indicated by red circles in Fig. 4e ) and Au(111) terraced substrate (yellow circles). The uniform diffraction pattern that appeared on the inch-scale sample should indicate the epitaxial growth of monolayer MoS 2 single crystal on the Au(223) facet (Fig. 4f and Supplementary Fig. 15 ). Fig. 4: Monolayer single-crystal MoS 2 films achieved by the growth and merging of monolayer MoS 2 ribbons. a Schematic illustration regarding the growth of monolayer MoS 2 single-crystal film through the merging of MoS 2 ribbons. Red and yellow spheres represent Mo and S atoms, respectively. b – d SEM images showing the growth process from narrow MoS 2 ribbons ( b ), wide ribbons ( c ), to continuous 2D film ( d ) by extending the growth time (t) from ∼ 2, ∼ 4, to ∼ 6 min, respectively. e Representative LEED pattern of monolayer MoS 2 single-crystal on the Au(223) facet. The spots indicated by red circles show the moiré satellite peaks for MoS 2 /Au(223). The spots indicated by yellow circles arise from the Au(111) facet. f More LEED patterns collected over an area of 10 mm × 4 mm. The red lines in the same direction indicate the same orientation of these patterns. g Low-magnification bright-field TEM image of a nearly full-coverage MoS 2 film transferred on the TEM grid. h Atomically resolved STEM image of the monolayer MoS 2 film, confirming its defect-free feature. i STEM images captured from the left and right edges of a monolayer MoS 2 ribbon presenting Mo-zz and S-zz edges, respectively. Full size image TEM and scanning transmission electron microscopy (STEM) characterizations were then conducted to identify the lattice orientation and edge structure. A representative atomically resolved STEM image presents well-ordered honeycomb lattices (Fig. 4h ). On large scales, the crystal lattice of MoS 2 maintains the same orientation, showing almost no obvious grain boundary. Selected-area electron diffraction (SAED) patterns collected on the film (Supplementary Fig. 16 ) reveal nearly identical lattice orientation (deviation smaller than ±0.1°), highly indicative of the single-crystal nature of the MoS 2 film. Moreover, the edge types on both sides of the monolayer MoS 2 ribbon are identified as Mo-zz and S-zz edges from both SAED pattern (Supplementary Fig. 17 ) and atomic-resolution STEM image (Fig. 4i ), and this result is consistent with our previous calculations. Dark-field TEM images of the monolayer MoS 2 film show uniform intensity over the entire area, again confirming its single crystallinity (Supplementary Fig. 18 ). On-site scanning tunneling microscopy (STM) measurements were then performed to determine the crystalline quality. A large-area STM image reveals the covering of a continuous monolayer MoS 2 film on the Au(111) terraces (Fig. 5a ). Further magnified image (from the region marked by the green square in Fig. 5a ) presents the evolution of a large-area hexagonally shaped moiré pattern with a period of ∼ 3.21 ± 0.10 nm (Fig. 5b ). Moreover, the orientation of the MoS 2 atomic row aligns well with the moiré row direction (as denoted by green and yellow arrows, respectively). This alignment was also confirmed by the corresponding 2D fast Fourier transform image (inset of Fig. 5b ), indicating an epitaxial relationship between them. As calculated, the moiré supercell (highlighted by a white rhombus) is in line with a (10 × 10) supercell of MoS 2 ( a 1 = 0.320 nm) on an (11 × 11) supercell of Au(111) ( a 2 = 0.288 nm). Furthermore, atomic-resolution STM images collected from the entire film show the same lattice orientation (Fig. 5b‒d and Supplementary Fig. 19 ), highly indicating the single-crystal nature of the monolayer MoS 2 film. Fig. 5: Single-crystal property characterizations of the continuous monolayer MoS 2 film achieved by the growth and merging of monolayer MoS 2 ribbons. a Large-area STM image ( V Tip = –0.61 V, I Tip = 3.55 nA) of the monolayer MoS 2 film on the Au(223) facet with Au(111) terrace. b Magnified STM image (–0.1 V, 30.77 nA) of the green square region in ( a ), presenting the perfect alignment of MoS 2 lattice direction with moiré row direction, as denoted by green and yellow arrows, respectively. Inset: corresponding 2D-FFT pattern. c , d Representative atomically resolved STM images of the moiré pattern for MoS 2 /Au(111), presenting a fixed period of ∼ 3.21 ± 0.10 nm (marked by white rhombus; −0.10 V, 40.95 nA; −0.1 V, 32.79 nA). e Photograph and corresponding OM image of a 1-inch single-crystal MoS 2 film transferred on SiO 2 /Si. f Raman mapping on the A 1g peak intensity for the monolayer MoS 2 single crystal showing a uniform color contrast. g PL mapping on the A exciton intensity of the monolayer film. h SHG mapping of the monolayer MoS 2 single crystal. Full size image Further photograph and optical microscopy (OM) images reveal homogenous color contrasts for the 1-inch single-crystal MoS 2 film transferred on SiO 2 /Si (Fig. 5e ). Additional Raman and PL intensity mappings also suggest the homogeneous optical properties (Fig. 5f, g ). Moreover, almost no obvious contrast difference can be noticed in the second-harmonic generation intensity mapping (Fig. 5h ), which unambiguously confirms the single crystallinity of the monolayer MoS 2 film. Syntheses of other monolayer TMDs ribbon arrays To further display the universality of our synthetic strategy, other TMDs ribbons and alloys, such as WS 2 , MoSe 2 , WSe 2 , and MoS x Se 2-x were also synthesized on the high-miller-index facets vicinal to Au(111) (Fig. 6a‒h ), by using MO 3 (M = Mo, W) and S, Se as precursors. Corresponding Raman data and STEM image confirm the desired chemical composition and monolayer nature of the ribbons. Fig. 6: Au-step-edge-directed growth of other monolayer TMDs ribbons. a , b . SEM image ( a ), representative Raman spectrum (inset of ( a )), and STEM image ( b ) of as-grown monolayer WS 2 ribbon arrays. c , d SEM image ( c ), representative Raman spectrum (inset of ( c )), and STEM image ( d ) of as-grown MoSe 2 ribbon arrays. e , f . SEM image ( e ), representative Raman spectrum (inset of ( e )), and STEM image ( f ) of as-grown monolayer WSe 2 ribbon arrays. g , h SEM image ( g ), representative Raman spectrum (inset of ( g )), and STEM image ( h ) of as-grown monolayer MoS x Se 2-x ribbon arrays. i AFM image of a representative monolayer MoS 2 ribbon-based device with a width of ~110 nm. j Output characteristics of the monolayer MoS 2 ribbon-based device. k Schematic illustration of the HER process. Red and yellow spheres represent Mo and S atoms, respectively, and the black dots denote the electric charges. l Tafel plots of the as-grown monolayer MoS 2 triangles and monolayer MoS 2 ribbons on Au/W electrodes. Full size image The ready access to monolayer TMDs ribbons provides us an opportunity for exploring their exotic electronic and catalytic performances. In order to characterize their electronic properties, back-gated FETs were constructed for MoS 2 ribbons on SiO 2 /Si substrates (Fig. 6i ). The transfer (Supplementary Fig. 20 ) and output curves (Fig. 6j ) of a representative device show typical n-type transfer characteristics. Statistical data measured on these FETs (Supplementary Fig. 21 ) show a narrow electron mobility distribution 7‒11 cm 2 V −1 s −1 and an on/off ratio of 10 5 ‒10 6 , comparable to the performance of 2D MoS 2 monolayers achieved on Au substrates [20] . Notably, the performance of the FETs based on monolayer MoS 2 grown on Au are not as good as those of monolayer MoS 2 films grown on sapphire [16] , [28] , [42] . This may originate from the different sample transfer processes used for them (e.g., electrochemical bubbling transfer), wherein contamination and structural defects were usually introduced. Hereby, a more efficient and clean sample transfer process should be developed in the future. Besides the potential application as channel material, monolayer MoS 2 ribbon was also predicted to possess higher catalytic performance in HER than its 2D counterpart, owing to the exposure of more abundant active edge sites. The applications of 1D monolayer MoS 2 ribbons and 2D monolayer MoS 2 flakes grown on Au/W substrates are also addressed as electrocatalysts in HER (Fig. 6k ). The overpotential (at a current density of 10 mA cm −2 ) and Tafel slope of monolayer MoS 2 ribbons were measured to be ~194 mV and 56 mV dec −1 , respectively, obviously lower than the values for 2D MoS 2 flakes (~220 mV and 71 mV dec −1 ) (Fig. 6l and Supplementary Fig. 22 ). Moreover, the catalytic current density exhibited negligible loss (<5%) after 1000 cycles, indicating the relatively high catalytic stability. The loading of the catalysts can be further increased toward low-cost, high-efficiency, and large-scale application explorations. In conclusion, we have realized the direct synthesis of periodic monolayer TMDs ribbon arrays, and wafer-scale TMDs single crystals on high-miller-index Au facets vicinal to (111) via a designed step-edge-directed synthetic strategy. Monolayer TMDs ribbons characterized by strictly monolayer thickness, high aspect ratio, relatively straight edge, and uniform alignment have been achieved. Based on this, an alternative epitaxial growth approach for wafer-scale TMDs single crystals is proposed by merging these uniformly aligned monolayer ribbons through a unique 1D edge-epitaxy mode. This work hereby opens a pathway for the single-crystal growth of 2D semiconductors on a wafer scale, as well as deepens our understanding of the epitaxial growth mechanism for the wafer-scale synthesis of 2D layered materials on insulating or conducting templates. This work should also propel the application explorations of monolayer TMDs ribbons or single crystals as channel materials in nanoelectronics and efficient catalysts in energy-related fields. Preparation of vicinal Au(111) single crystals The commercial polycrystalline gold foils (99.99%, ~50 µm thickness) were first ultrasonic cleaned in HCl solution (20% wt) for 10 min, and then in an acetone solution for 10 min. To prepare the high-miller-index facets vicinal to Au(111), a piece of cleansed gold foil was placed on an etched tungsten foil on a graphite boat, annealing at ~1100 °C for 20 min with a mixture of Ar/H 2 (300/50 sccm) as the carrier gas. The gold will firstly melt into liquid at ~1100 °C, and resolidified to induce the formation of Au(111) vicinal facets after cooling down processes. Synthesis of monolayer TMDs ribbons For the growth of MoS 2 ribbons, the MoO 3 and S powders were placed in the upstream of Au(111)/W substrate at a distance of 4 and 20 cm in a three-zone tube furnace, respectively. The growth was performed in a low-pressure environment with the protection of Ar (50 sccm) gas. The typical temperatures of S, MoO 3 (2‒3 mg), and Au(111) substrates were ~100, ~530, and ~750 °C, respectively. The S/Mo ratio was defined by the quantity of S and MoO 3 precursors. Notably, this growth temperature was relatively higher than that used for the growth of triangular monolayer MoS 2 domains (~720 °C) in our previous work [20] . For the growth of monolayer WS 2 ribbons, the typical temperatures of S, WO 3 , and Au substrates were set at ~100, 820, and 820 °C, respectively. For the growth of 1D monolayer MoSe 2 and WSe 2 ribbons, a mixture of Ar (50 sccm) and H 2 (5 sccm) was used as the carrier gas. The Se powder was placed in the upstream of a substrate at a distance of 16 cm. The typical temperatures for Se, MoO 3 (WO 3 ), and Au substrates were set at ~200, 530 (820), 820 °C, respectively. For the synthesis of monolayer MoS x Se 2– x ribbons, the MoO 3 precursor and a mixed S and Se precursor were placed in the upstream of Au/W substrate at a distance of 1 and 20 cm, respectively. The typical temperatures for the Au substrates, MoO 3 , and S/Se mixture were set at 850, 800, and 200 °C, respectively. The growth process was performed under a mixture flow of Ar (50 sccm) and H 2 (5 sccm) gases. The synthetic recipes for MoS 2 ribbons grown on graphene and h -BN monolayers are provided in the Supplementary information. Calculation methods The theoretical calculations based on DFT were performed by the Vienna ab initio simulation package [43] . Details of calculations are provided in the Supplementary information. Characterization of MoS 2 ribbons The MoS 2 ribbons and single crystals were systematically characterized by SEM (Hitachi S-4800, 2 kV), OM (Nikon ECLIPSE, LV100ND), Raman and PL spectroscopy (Horiba Jobin-Yvon, LabRAM HR800, with an excitation wavelength of 532 nm), spectral imaging (WITec, Alpha 300R), AFM (Bruker, Dimension Icon), XPS (Kratos Analytical Ltd. AXIS-Ultra with monochromatic Al Ka X-ray), TEM (FEI Tecnai F20, acceleration voltage of 200 kV), STEM (JEOL ARM200F, acceleration voltage 80 kV), and STM (Omicron, the base pressure: 10 −10 mbar). 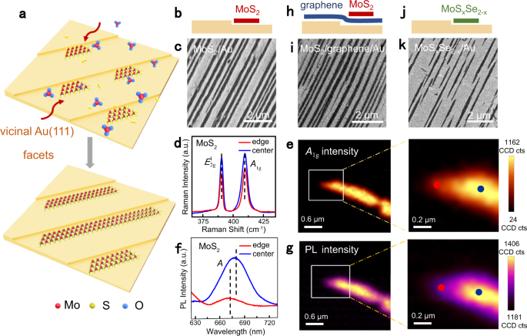Fig. 2: Universal growth of aligned monolayer TMDs ribbons along the step edges of Au(111) vicinal facets. aSchematic illustration of the growth of well-aligned monolayer MoS2ribbons along the step edges of vicinal Au(111) facets. The red, yellow, and blue spheres represent Mo, S, and O atoms, respectively, and the red arrows indicate the diffusion pathways of the active species.b,cSchematic side view and SEM image of aligned monolayer MoS2ribbons grown on Au(223) facet, respectively.dRepresentative Raman spectra of the edges (red) and centers (blue) of monolayer MoS2ribbons transferred on SiO2/Si substrates.eRaman mapping on the intensity ofA1gpeak for a MoS2ribbon. The right panel is the magnified image of the white rectangle marked region in the left panel. The red and blue dots mark the edge and center positions of MoS2ribbon, respectively. a.u., arbitrary units.f,gRepresentative PL spectra of the edges (red) and centers (blue) of a MoS2ribbon and its PL mapping on the intensity of A peak. The right panel is the magnified image of the white rectangle marked region in the left panel. The red and blue dots in (g) mark the edge and center positions of MoS2ribbon, respectively.h,iSchematic side view and SEM image of monolayer MoS2ribbons grown on monolayer graphene covered Au(213) facet, respectively.j,kSchematic side view and SEM image of monolayer MoSxSe2-xribbons grown along the steps of Au(235) facet, respectively. The LEED measurements were carried out in an ultra-high vacuum (3 × 10 −10 Torr) and the electron energy was fixed at 96 eV. 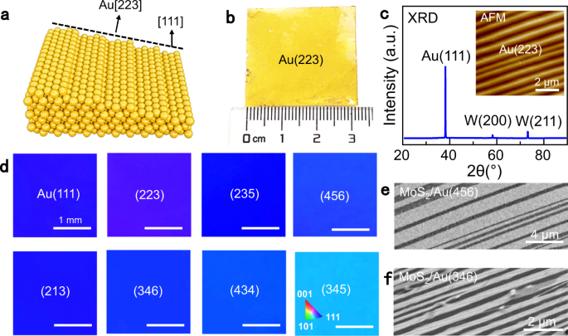Fig. 3: Preparation of inch-scale high-miller-index Au single-crystal films (Au(111) vicinal facets). aSchematic illustration of a high-index Au(223) facet.bRepresentative photography of the evolved Au(223) single-crystal film on the W template.c. XRD pattern of Au/W foils showing the evolution of single-crystal Au(111) film. Inset: AFM image of a single-crystal Au film with Au(223) facet.dRepresentative EBSD IPF maps of the as-prepared Au films, with crystal facets of (111), (223), (235), (456), (213), (346), (434), (345), respectively. The scale bars in all panels are 1 mm.e,fSEM images of the unidirectionally aligned monolayer MoS2ribbons evolved on single-crystal Au(456) (e) and Au(346) (f), respectively. 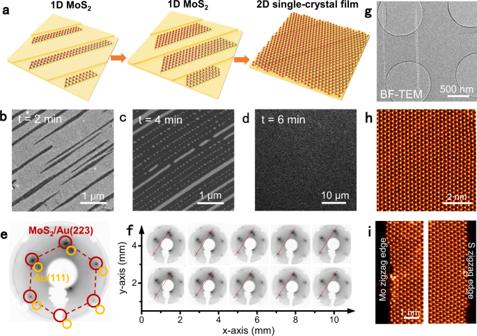Fig. 4: Monolayer single-crystal MoS2films achieved by the growth and merging of monolayer MoS2ribbons. aSchematic illustration regarding the growth of monolayer MoS2single-crystal film through the merging of MoS2ribbons. Red and yellow spheres represent Mo and S atoms, respectively.b–dSEM images showing the growth process from narrow MoS2ribbons (b), wide ribbons (c), to continuous 2D film (d) by extending the growth time (t) from∼2,∼4, to∼6 min, respectively.eRepresentative LEED pattern of monolayer MoS2single-crystal on the Au(223) facet. The spots indicated by red circles show the moiré satellite peaks for MoS2/Au(223). The spots indicated by yellow circles arise from the Au(111) facet.fMore LEED patterns collected over an area of 10 mm × 4 mm. The red lines in the same direction indicate the same orientation of these patterns.gLow-magnification bright-field TEM image of a nearly full-coverage MoS2film transferred on the TEM grid.hAtomically resolved STEM image of the monolayer MoS2film, confirming its defect-free feature.iSTEM images captured from the left and right edges of a monolayer MoS2ribbon presenting Mo-zz and S-zz edges, respectively. 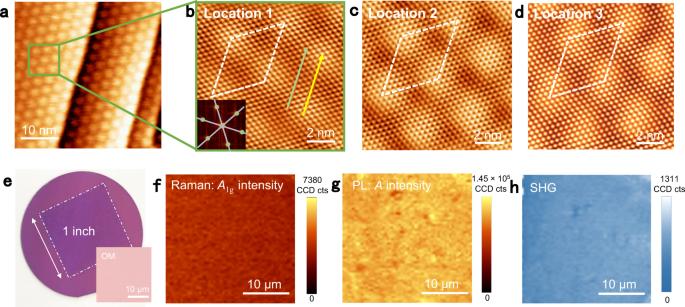Fig. 5: Single-crystal property characterizations of the continuous monolayer MoS2film achieved by the growth and merging of monolayer MoS2ribbons. aLarge-area STM image (VTip= –0.61 V,ITip= 3.55 nA) of the monolayer MoS2film on the Au(223) facet with Au(111) terrace.bMagnified STM image (–0.1 V, 30.77 nA) of the green square region in (a), presenting the perfect alignment of MoS2lattice direction with moiré row direction, as denoted by green and yellow arrows, respectively. Inset: corresponding 2D-FFT pattern.c,dRepresentative atomically resolved STM images of the moiré pattern for MoS2/Au(111), presenting a fixed period of∼3.21 ± 0.10 nm (marked by white rhombus; −0.10 V, 40.95 nA; −0.1 V, 32.79 nA).ePhotograph and corresponding OM image of a 1-inch single-crystal MoS2film transferred on SiO2/Si.fRaman mapping on theA1gpeak intensity for the monolayer MoS2single crystal showing a uniform color contrast.gPL mapping on theAexciton intensity of the monolayer film.hSHG mapping of the monolayer MoS2single crystal. 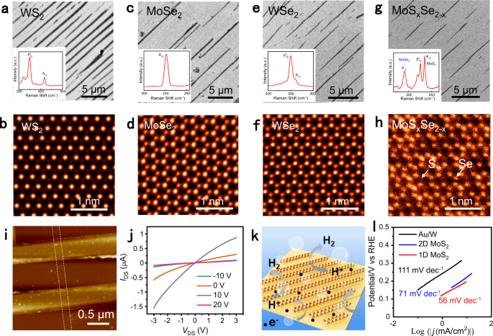Fig. 6: Au-step-edge-directed growth of other monolayer TMDs ribbons. a,b. SEM image (a), representative Raman spectrum (inset of (a)), and STEM image (b) of as-grown monolayer WS2ribbon arrays.c,dSEM image (c), representative Raman spectrum (inset of (c)), and STEM image (d) of as-grown MoSe2ribbon arrays.e,f. SEM image (e), representative Raman spectrum (inset of (e)), and STEM image (f) of as-grown monolayer WSe2ribbon arrays.g,hSEM image (g), representative Raman spectrum (inset of (g)), and STEM image (h) of as-grown monolayer MoSxSe2-xribbon arrays.iAFM image of a representative monolayer MoS2ribbon-based device with a width of ~110 nm.jOutput characteristics of the monolayer MoS2ribbon-based device.kSchematic illustration of the HER process. Red and yellow spheres represent Mo and S atoms, respectively, and the black dots denote the electric charges.lTafel plots of the as-grown monolayer MoS2triangles and monolayer MoS2ribbons on Au/W electrodes. The electron beam spot size is about 500 μm. The single-crystal Au(111) vicinal facets were characterized by XRD (Bruker D8-Discover, with a Cu Kα radiation source) and EBSD (Oxford instruments).